Unconventional molecule-resolved current rectification in diamondoid–fullerene hybrids The unimolecular rectifier is a fundamental building block of molecular electronics. Rectification in single molecules can arise from electron transfer between molecular orbitals displaying asymmetric spatial charge distributions, akin to p–n junction diodes in semiconductors. Here we report a novel all-hydrocarbon molecular rectifier consisting of a diamantane–C 60 conjugate. By linking both sp 3 (diamondoid) and sp 2 (fullerene) carbon allotropes, this hybrid molecule opposingly pairs negative and positive electron affinities. The single-molecule conductances of self-assembled domains on Au(111), probed by low-temperature scanning tunnelling microscopy and spectroscopy, reveal a large rectifying response of the molecular constructs. This specific electronic behaviour is postulated to originate from the electrostatic repulsion of diamantane–C 60 molecules due to positively charged terminal hydrogen atoms on the diamondoid interacting with the top electrode (scanning tip) at various bias voltages. Density functional theory computations scrutinize the electronic and vibrational spectroscopic fingerprints of this unique molecular structure and corroborate the unconventional rectification mechanism. Following their discovery about a quarter-century ago [1] , fullerenes attracted considerable attention for their fascinating geometry and have since become emblematic elements in the fabrication of complex ensembles of organized nanostructures [2] , [3] , [4] , [5] . Their electronic properties, ranging from semiconductivity to superconductivity [6] , [7] , have spurred the search for derivatives encoding information stored in the arrangement of suitable binding sites, and for switching and reading out this information through interactions. Despite intensive efforts [8] , [9] , [10] , the integration of fullerenes with other carbon allotropic forms and the identification of dynamic features for the controlled electromechanical switching between different superstructural arrangements remains considerably challenging. Diamondoids [11] , [12] have intrinsic capabilities of self-assembly and electron transfer and therefore represent attractive candidates for building nanostructured materials, such as monochromatic high-efficiency field emitters [13] or robust mechanical coatings. Additional features—including molecular geometries, selective functionalization and stacking interactions—enable the emergence of singular electronic phenomena in topologically favoured architectures [14] , [15] . The development of large-area molecular devices has been established as an important area in nanoscience and nanotechnology applications, merging bottom-up self-assembly techniques with massively parallel architectures and fault-tolerant algorithms [16] . Fostered by pioneering work of Aviram and Ratner [17] , rectification in single molecules typically involves electron transfer between molecular orbitals displaying asymmetric probability amplitudes. This general mechanism has been applied to understanding rectification arising from electron tunnelling through molecular [18] and supramolecular components [19] . Here, we demonstrate that diamondoid properties can be readily transcribed into molecular rectifiers by their advantageous coupling with fullerenes via synthetic techniques. Accordingly, we probed by low-temperature scanning tunnelling microscopy (STM) and spectroscopy (STS) the morphology and conductance of various self-assembled diamantane–C 60 domains deposited at room temperature on Au(111) from diluted toluene solutions. Our data reveal an intriguing rectifying behaviour within the molecular constructs. This unconventional electronic behaviour likely originates from the electrostatic repulsion of Dia–C 60 molecules due to the interaction of positively charged terminal hydrogen atoms on the diamondoid with the scanning tip at various bias voltages, in agreement with charge density values estimated on the Dia–C 60 hybrid molecule by density functional theory (DFT) calculations. Design and synthesis of the diamondoid–fullerene molecule In an effort to design novel rectification-capable molecules, the diamantane–fullerene combination was selected because of the optimal energy level configurations displayed by these two carbon structures ( Supplementary Fig. 1 ). More specifically, the lowest unoccupied molecular orbital (LUMO) of C 60 lines up closer to the Fermi level of the metallic substrates than does its highest occupied molecular orbital (HOMO). Seminal optical absorption measurements [20] revealed that the opposite holds for diamantane. This suggests that diamantane–C 60 (Dia–C 60 ) hybrid molecules should be ideal molecular rectifiers by combining a negative electron affinity moiety (localized on diamantane) with a positive electron affinity segment (localized on C 60 ). Since C 60 —noble metal electrode interfaces exhibit reduced variability in transport characteristics [21] , gold substrates are a suitable choice for examining the electronic performance of the physisorbed Dia–C 60 conjugate. The 2-(diamant-4-yl)butadiene-1,3-C 60 adduct (Dia–C 60 ) was synthesized through thermal Diels–Alder reaction of 4-butadienyl diamantane and C 60 in 84% yield [22] . The DFT-computed average orbital density for the isolated Dia–C 60 construct along the molecular axis versus energy is shown in Fig. 1a (see also the Methods Section and Suplementary Information, Supplementary Fig. 1 ). The resulting integrated projected density of states plot reveals the segregation of both diamantane- and C 60 -like energy levels on the two opposite ends of the molecule axis, and a negligible overlap across the cyclohexene linker. While this is an essential requirement for efficient molecular rectifiers, the energy levels do not simply conform to the donor–acceptor convention proposed by Aviram and Ratner [17] , namely, the C 60 -like states (acceptor states) lie entirely within the band-gap of the diamondoid-like states (donor states), rather than being offset from them. Hence, we do not expect the Dia–C 60 molecules to behave as conventional Aviram–Ratner rectifiers. 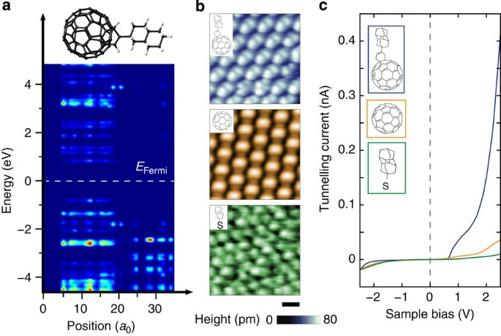Figure 1:Energy diagram of Dia–C60and comparison with constituent molecules. (a) Colour map of the projected density of states of the Dia–C60molecule integrated over thex–yplane as a function of thez-coordinate (molecular axis, in units of the Bohr radiusa0) and energy. The Fermi energy of the Dia–C60on Au(111) system is indicated by the dashed white line. To account for the HOMO–LUMO energy underestimation within DFT, a scissors operator (rigid shift) has been applied to correct the HOMO–LUMO separation. (b) 5 × 5 nm2STM images of Dia–C60(I=20 pA,V=2.5 V, top row), C60(I=200 pA,V=2.5 V, middle row) and diamantane-4-thiol (I=20 pA,V=2.0 V, bottom row) covering Au(111) substrates. Scale bar, 1 nm. (c) Current–voltage spectra measured on the adlayers illustrated inb. Tunnelling conditions for all measurements areI=20 pA andV=−2.5 V. Each curve corresponds to the average of a dozen of individualI–Vtraces measured over the centres of various molecules in the adlayers. Figure 1: Energy diagram of Dia–C 60 and comparison with constituent molecules. ( a ) Colour map of the projected density of states of the Dia–C 60 molecule integrated over the x–y plane as a function of the z -coordinate (molecular axis, in units of the Bohr radius a 0 ) and energy. The Fermi energy of the Dia–C 60 on Au(111) system is indicated by the dashed white line. To account for the HOMO–LUMO energy underestimation within DFT, a scissors operator (rigid shift) has been applied to correct the HOMO–LUMO separation. ( b ) 5 × 5 nm 2 STM images of Dia–C 60 ( I =20 pA, V =2.5 V, top row), C 60 ( I =200 pA, V =2.5 V, middle row) and diamantane-4-thiol ( I =20 pA, V =2.0 V, bottom row) covering Au(111) substrates. Scale bar, 1 nm. ( c ) Current–voltage spectra measured on the adlayers illustrated in b . Tunnelling conditions for all measurements are I =20 pA and V =−2.5 V. Each curve corresponds to the average of a dozen of individual I–V traces measured over the centres of various molecules in the adlayers. Full size image Rectification and contrast with molecular constituents The prominent submolecular features expressed by the Dia–C 60 molecular arrays on the Au(111) surface are highlighted in Fig. 1b , in comparison with the hexagonal molecular arrangement of bare C 60 , and the denser diamantane-thiol self-assembled monolayers (SAMs) on gold substrates. Careful STM and STS studies of these SAM systems prove that the electronic behaviour of the Dia–C 60 hybrid molecule is more complex than the sum of its constituents. Figure 1c presents the asymmetric electrical current ( I ) versus bias voltage ( V ) response of Dia–C 60 , contrasting sharply with the recorded spectroscopic I–V characteristics for the individual C 60 and diamantane-4-thiol species. Topographical structure of molecular monolayers A long-range topograph spanning multiple Dia–C 60 domains is presented in Fig. 2a . An ordered two-dimensional lattice of Dia–C 60 molecules is visible, as well as a seemingly disordered low-conductance region (dark-blue areas). Point-like defects consisting of missing single or few molecules are common, and affect 20±4% of the lattice sites. This molecular arrangement differs from the regular C 60 SAM (inset to Fig. 2a ), which essentially displays full coverage. Despite this decrease in coverage, the estimated lattice constant of 9.5±0.3 Å for the Dia–C 60 SAM is close to the measured C 60 spacing of 9.8±0.2 Å, both of which corroborate the ≈1.0 nm value reported in the literature [3] , [23] . Thus, we infer that the diamantane moiety is nearly vertically oriented in Dia–C 60 adsorbed on Au(111) substrates, suggesting a generic hosting property of other metallic surfaces for Dia–C 60 molecules. The low coverage of Dia–C 60 indicates that the presence of the diamondoid alters the delicate equilibrium between the fullerene–surface and molecule–molecule interactions responsible for producing high-coverage SAMs. We attribute the low-conductance regions to disordered, prostrate Dia–C 60 molecules (or fragments thereof), or solvent molecules that are not displaced by the Dia–C 60 during SAM formation. In some areas, the low-conductance regions exhibit self-assembled domains of toluene molecules (see insets to Fig. 2b ). This is likely a byproduct of the long-range physisorption of the Dia–C 60 dyads on gold surfaces, further evidencing the fact that the diamondoid–fullerene lattice is less stable than that of C 60 , for which no self-organized toluene or low-conductance regions were detected. The possiblity that the toluene layer exists underneath the Dia–C 60 lattice can be ruled out for a number of reasons. If the molecular arrangement of Dia–C 60 on toluene was stable on Au(111), we would expect at least a coverage-dependent formation of different toluene and paired Dia–C 60 on toluene domains for various self-assembly times. Instead, increasing the exposure time of the gold substrates to the molecular solution negligibly improves the overall Dia–C 60 coverage. Second, we would predict some of the isolated Dia–C 60 molecules lying on toluene—which can easily be identified spectroscopically—to have the same height as those in the Dia–C 60 lattice, which we do not observe ( Fig. 2b ). Finally, neighbouring strips of toluene rows caused by the Au(111) herringbone reconstruction are offset from one another by half the width of a toluene row, whereas the Dia–C 60 lattice extends without defect over the length scale of the herringbone pattern. 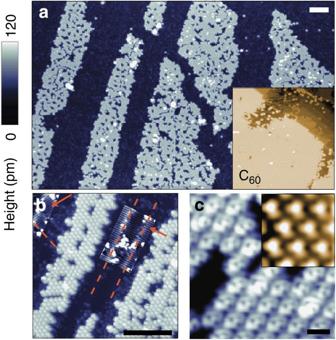Figure 2:STM images displaying the packing and structure of Dia–C60adlayers. (a) Long-range 160 × 100 nm2STM image of hexagonally packed Dia–C60molecules on Au(111) with 42±3% coverage (I=20 pA,V=2.5 V). Inset: for reference, C60hexagonally packed on Au(111) with nearly 100% coverage (I=100 pA,V=2.0 V). Same scale as in the Dia–C60topography imagea. Scale bar, 10 nm. (b) A 30 × 30-nm2topography image of Dia–C60molecules on Au(111). Dark regions outside the two domains are covered by toluene molecules organized in stripes. Contrast in boxed regions is enhanced to make toluene stripes (orange arrows) and the underlying Au(111) herringbone reconstruction (dashed orange lines) visible. Scale bar, 10 nm. (c) A 6.5 × 6.5-nm2topography image of Dia–C60molecules on Au(111) showing the submolecular structure (I=20 pA,V=−2.5 V). Inset: zoom into the C60adlayer (I=100 pA,V=−2.5 V). Inset is same scale as main imagec. Scale bar, 1 nm. At this particular bias voltage, C60molecules exhibit threefold symmetry, whereas Dia–C60dyads do not. Figure 2: STM images displaying the packing and structure of Dia–C 60 adlayers. ( a ) Long-range 160 × 100 nm 2 STM image of hexagonally packed Dia–C 60 molecules on Au(111) with 42±3% coverage ( I =20 pA, V =2.5 V). Inset: for reference, C 60 hexagonally packed on Au(111) with nearly 100% coverage ( I =100 pA, V =2.0 V). Same scale as in the Dia–C 60 topography image a . Scale bar, 10 nm. ( b ) A 30 × 30-nm 2 topography image of Dia–C 60 molecules on Au(111). Dark regions outside the two domains are covered by toluene molecules organized in stripes. Contrast in boxed regions is enhanced to make toluene stripes (orange arrows) and the underlying Au(111) herringbone reconstruction (dashed orange lines) visible. Scale bar, 10 nm. ( c ) A 6.5 × 6.5-nm 2 topography image of Dia–C 60 molecules on Au(111) showing the submolecular structure ( I =20 pA, V =−2.5 V). Inset: zoom into the C 60 adlayer ( I =100 pA, V =−2.5 V). Inset is same scale as main image c . Scale bar, 1 nm. At this particular bias voltage, C 60 molecules exhibit threefold symmetry, whereas Dia–C 60 dyads do not. Full size image High-resolution topographs over Dia–C 60 and C 60 molecules reveal bias-dependent submolecular-scale features ( Fig. 2c ). The well-known threefold and twofold symmetry patterns—visible in the C 60 SAMs on Au(111) at negative and positive V , respectively—are reduced in the Dia–C 60 SAM because of the diamondoid. Indeed, the effect of the diamondoid’s presence on the topographic appearance of the fullerene-derivative adlayer is especially perceptible at V =−2.5 V ( Fig. 2c , lower left), where a protrusion is visible in the lower left of each molecule. This eccentric asymmetry matches the calculated projected density of states ( Supplementary Fig. 1 ), since the dominant contribution of the diamondoid in the electronic states is found to occur at approximately −2.0 eV below the Fermi level. The unoccupied states ( V >0) present minor variations compared with the C 60 states, both exhibiting a two-lobed shape, although a more submolecular structure can be observed on the Dia–C 60 topographs (that is, lower symmetry), presumably due to the lifted degeneracy caused by the chemical bonding of the diamondoid ( Supplementary Figs 1–3 ). Electronic spectroscopy of single molecules We now turn to the electronic properties of the individual Dia–C 60 molecules. The I–V curve and the dI/dV spectrum recorded over the centre of a Dia–C 60 molecule are shown in Fig. 3a,b , along with typical C 60 measurements. In these measurements, the bias voltage has been set to V =+2.5 V (compared with −2.5 V in Fig. 1a ) to prevent saturation of the lock-in detector used to measure dI/dV ; the rectification is therefore manifested in these measurements as a decrease in the Dia–C 60 current (relative to C 60 ) for V <0, rather than an increase in current for V >0. Similarities are readily apparent between the STS spectra of Dia–C 60 and C 60 , namely, local maxima in dI/dV traces at voltages corresponding to the energies of the bare C 60 HOMO, LUMO and LUMO+1 states (compare with Supplementary Fig. 1a,c ). The amplitude of the Dia–C 60 conductance in the occupied states ( V <0) is, however, noticeably reduced compared with C 60 . Interestingly, the strongly asymmetric current in the Dia–C 60 molecule arises in the opposite bias direction than the Aviram–Ratner effect predicts. For the particular I–V curve discussed here, the Dia–C 60 allows the passage of ~6.5 times more current at 2.5 V than at −2.5 V, while the C 60 displays a rectification ratio of only 2.2 (where rectification ratio R is defined as | I ( V )/ I (− V )| at V =2.5 V). We find the conductance suppression at negative V— and the resulting asymmetric I–V curve—to be the norm across many distinctive molecules, domains and samples. The resulting rectification behaviour reflects the qualitatively equivalent current–voltage data taken during spectroscopy in both positive to negative and reverse bias sweep directions ( Figs 1 and 3 ). Its emergence alludes to the subtle role the diamondoid plays by contributing to the unoccupied molecular states of Dia–C 60 , which are located in close proximity of the Fermi level and, spatially, near the tip (see Fig. 1a ). 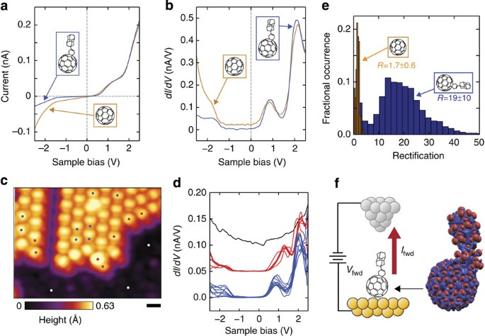Figure 3:Single-moleculeI–VanddI/dVmeasurements and histogram of rectification factors at 4.5 K. (a)I–Vmeasurements over Dia–C60(blue) and C60(orange) molecules highlighting their spectral similarity at positive bias and the suppression of conductance at negative bias for the Dia–C60dyad. (b)dI/dVpoint-spectra over the Dia–C60molecule (blue) and the C60molecule (orange) collected simultaneously with theI–Vcurves shown ina. (c) Region with Dia–C60molecules over which the spectra shown indwere recorded. Dots in the adlayer represent the location of individual point-spectra, with colours corresponding to thedI/dVspectra colours: blue refers to the middle of the lattice (six nearest neighbours) and red refers to the edge of the lattice (<6 nearest neighbours). Scale bar, 1 nm. (d) For reference, the black trace is the average of the spectra taken over the white dots inc, located in a disordered sample area, and it has been shifted for clarity. The tunnelling junction was stabilized atV=2.5 V before turning the feedback off and performing the measurements:I=200 pA (a,b) and 100 pA ind. (e) Distribution of the rectification factors determined at ±2.5 V for Dia–C60(blue) and C60(orange). (f) Sketch shows the orientation of the Dia–C60on the gold surface and the direction of forward bias. Electronic charge density differences in an isolated Dia–C60molecule where subtraction of each atomic contribution has been applied. This electronic density distribution provides information regarding the chemical behaviour of the Dia–C60dyad, where the negative charge (blue) is more spatially localized on the C60while the positive charge (red) is predicted closer to the diamantane moiety. Positive and negative electronic density isosurfaces correspond to ±0.05 electron Å−3, respectively. Figure 3c,d illustrates how STS measurements are observed to vary between different individual molecules. On one hand, the blue curves in Fig. 3d were all measured over molecules with six nearest neighbours, and all exhibit C 60 -like HOMO, LUMO and LUMO+1 peaks. On the other hand, STS measurements on molecules occupying the edge of the two-dimensional lattice (red curves in Fig. 3d ) present an increase in the energy of the C 60 -like LUMO peak of ~0.3 eV. This effect has been previously observed in C 60 adlayers [24] , and has been attributed to differences in the intramolecular screening occurring at the edge of the lattice. The fact that a similar effect is observed in our diamantane–fullerene samples points out that the intramolecular interactions seen in C 60 adlayers are likewise present in Dia–C 60 lattices. Figure 3: Single-molecule I–V and dI/dV measurements and histogram of rectification factors at 4.5 K. ( a ) I–V measurements over Dia–C 60 (blue) and C 60 (orange) molecules highlighting their spectral similarity at positive bias and the suppression of conductance at negative bias for the Dia–C 60 dyad. ( b ) dI/dV point-spectra over the Dia–C 60 molecule (blue) and the C 60 molecule (orange) collected simultaneously with the I–V curves shown in a . ( c ) Region with Dia–C 60 molecules over which the spectra shown in d were recorded. Dots in the adlayer represent the location of individual point-spectra, with colours corresponding to the dI/dV spectra colours: blue refers to the middle of the lattice (six nearest neighbours) and red refers to the edge of the lattice (<6 nearest neighbours). Scale bar, 1 nm. ( d ) For reference, the black trace is the average of the spectra taken over the white dots in c , located in a disordered sample area, and it has been shifted for clarity. The tunnelling junction was stabilized at V =2.5 V before turning the feedback off and performing the measurements: I =200 pA ( a , b ) and 100 pA in d . ( e ) Distribution of the rectification factors determined at ±2.5 V for Dia–C 60 (blue) and C 60 (orange). ( f ) Sketch shows the orientation of the Dia–C 60 on the gold surface and the direction of forward bias. Electronic charge density differences in an isolated Dia–C 60 molecule where subtraction of each atomic contribution has been applied. This electronic density distribution provides information regarding the chemical behaviour of the Dia–C 60 dyad, where the negative charge (blue) is more spatially localized on the C 60 while the positive charge (red) is predicted closer to the diamantane moiety. Positive and negative electronic density isosurfaces correspond to ±0.05 electron Å −3 , respectively. Full size image The rectification ratio has been determined for ~10 3 individual I–V measurements recorded over Dia–C 60 molecules. A histogram of these results is shown in Fig. 3e together with a histogram computed from 200 measurements taken on a C 60 monolayer. The particular electronic structure of the Dia–C 60 molecule enables one order of magnitude higher average rectification. Reports of unimolecular rectification in the literature vary widely, spanning a range from slightly greater than unity to higher than 1,000, and are typically reported for voltages up to 3 V (ref. 18 ). These values come from single-molecule measurements in STM or break-junction geometries as well as measurements of thin layers with conducting atomic force microscopy probes and large-area devices with molecular tunnelling junctions [19] . The Dia–C 60 molecule represents to our knowledge the first molecular rectifier that is a pure hydrocarbon, pairs two molecules displaying negative and positive electron affinities, respectively, and combines a caged sp 3 molecule with a spherical sp 2 network. Vibrational spectroscopy of single molecules Additional insight into the transport mechanisms responsible for unimolecular rectification can be obtained via vibronic spectroscopy [14] , [25] , [26] , [27] , [28] . The presence of inelastic modes in molecule-adsorbed metallic surfaces can be detected as anti-symmetric peaks in d 2 I/dV 2 spectra [29] . Low-bias spectroscopy reveals a distinct signature of such modes over the Dia–C 60 adlayer ( Fig. 4a ). The d 2 I/dV 2 peak at 57 mV is only present over the Dia–C 60 molecules, indicating that we are exciting vibrational modes localized to the hybrid construct. To understand this spectroscopic feature, the vibrational spectrum of the Dia–C 60 molecule has been computed using DFT and compared with the C 60 spectrum in the corresponding energy range. A series of low-frequency modes in the vicinity of 57 meV can be observed in Fig. 4b , resulting in a peak in the phonon spectrum closely matching the spectroscopy data. Most of these vibrational modes involve all the atomic constituents of the Dia–C 60 hybrid, although a few of them correspond to localized atomic motions in the diamantane structure ( Fig. 4c ; Supplementary Fig. 4 ). Indeed, Li et al. [30] recently highlighted the softening of the vibrational modes at metal–C 60 interfaces due to both external electric fields, and doping or charge transfer. Similarly, the C 60 –dia molecule exhibiting a covalent binding between the two components reveals at low energies a strong coupling between the respective vibration modes. The DFT computations provide further evidence for the diamondoid-up structural orientation, as tunnelling electrons should couple most strongly to vibrational modes located on the part of the molecule closest to the tip. 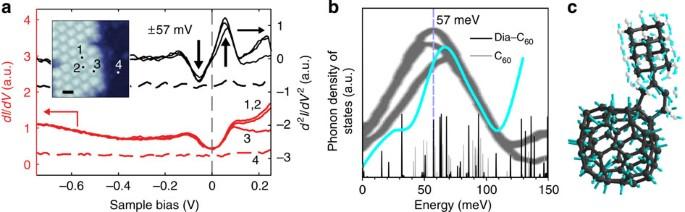Figure 4:Low-voltage inelastic tunnelling spectroscopy and computed dynamical properties in Dia–C60. (a)dI/dV(red, left axis) andd2I/dV2(black, right axis) measurements of Dia–C60molecules in an adlayer and the adjacent disorder area (I=100 pA,V=−0.75 V) at 4.5 K. The curves were recorded at the locations indicated in the inset. Scale bar, 1 nm. Solid curves (1–3) were measured over the Dia–C60molecules and display anti-symmetric peaks at ±57 meV, whereas the dashed trace (4) was collected over the disordered region. (b) Phonon density of states of Dia–C60(black spectrum) and C60(light-grey spectrum) molecules. The background image is thed2I/dV2curve already illustrated ina. The cyan curve is the computed Dia–C60phonon spectrum with a 20 meV broadening chosen to match the experimentally observed linewidths. The dashed line indicates the centre of thed2I/dV2peak at 57 meV, which corresponds to a phonon mode illustrated incby the arrows in the ball-and-stick Dia–C60model. Most phonon modes within the 50–70 meV range involve vibrations of the whole molecule. (c) The 57 meV vibrational mode of the hybrid molecule is displayed with the ball-and-stick Dia–C60model. Figure 4: Low-voltage inelastic tunnelling spectroscopy and computed dynamical properties in Dia–C 60 . ( a ) dI/dV (red, left axis) and d 2 I/dV 2 (black, right axis) measurements of Dia–C 60 molecules in an adlayer and the adjacent disorder area ( I =100 pA, V =−0.75 V) at 4.5 K. The curves were recorded at the locations indicated in the inset. Scale bar, 1 nm. Solid curves (1–3) were measured over the Dia–C 60 molecules and display anti-symmetric peaks at ±57 meV, whereas the dashed trace (4) was collected over the disordered region. ( b ) Phonon density of states of Dia–C 60 (black spectrum) and C 60 (light-grey spectrum) molecules. The background image is the d 2 I/dV 2 curve already illustrated in a . The cyan curve is the computed Dia–C 60 phonon spectrum with a 20 meV broadening chosen to match the experimentally observed linewidths. The dashed line indicates the centre of the d 2 I/dV 2 peak at 57 meV, which corresponds to a phonon mode illustrated in c by the arrows in the ball-and-stick Dia–C 60 model. Most phonon modes within the 50–70 meV range involve vibrations of the whole molecule. ( c ) The 57 meV vibrational mode of the hybrid molecule is displayed with the ball-and-stick Dia–C 60 model. Full size image The unique structure of the diamantane–fullerene dyad potentially facilitates an unconventional operation for the molecular rectifier. This rectification mechanism relies on the presence of the hydrogen atoms at the diamondoid surface that are partially positively charged, as illustrated in Fig. 3f . When a positively biased tip ( V <0) is brought close to the tip of the molecule, we expect the positively charged hydrogen atoms to be repelled by the tip. Accordingly, the top part of the molecule rotates away from the tip. In the case of STM measurements, this effect would cause the current to decrease (due to increased tip–molecule distance) whenever the tip bias becomes more positive at constant height—as in dI/dV spectroscopy. As a result, the current would be reduced when the sample bias sweeps from positive to negative, producing a rectifying effect consistent with the observed behaviour shown in Fig. 3a . This type of molecular motion could be related to the inelastic tunnelling signature observed in Fig. 4 , especially since it is suggestive of a high degree of motion of the diamondoid. Indeed, this field-induced motion effect could be observed in these fullerene derivatives because of the subtle intramolecular dynamics of the hydrogen-terminated diamantane interacting with the tip electrode. In summary, we demonstrate that the low-temperature I–V characteristics of a diamondoid–fullerene hybrid molecule, probed by scanning tunnelling spectroscopy, are strikingly different than those of its constituents. The Dia–C 60 dyads essentially display a C 60 -like spectrum in which tunnelling through the occupied states is suppressed, while the through-molecule tunnelling process seems influenced by diamondoid molecular motions that remain unconstrained in the ordered assemblies. This work can be further exploited to design novel hydrocarbon-based single-molecule rectifiers. Materials Synthesis of 2-(diamant-4-yl)butadiene-1,3-C 60 adduct ( Dia–C 60 ): a mixture of 0.1 g (0.140 mmol) of fullerene C 60 and 34 mg (0.140 mmol) of 2-(diamant-4-yl)butadiene prepared as previously described [22] was refluxed under argon in 100 ml of dry toluene for 4.5 h. Excess solvent was evapourated; the remainder was dissolved in CS 2 mixed with 15 ml of pentane and stirred at room temperature for 10 min, filtered, washed with pentane, dried in vacuo and stored dry to give 112 mg (84%) of a cherry-brown powder. 1 H NMR ( δ , CDCl 3 ): 6.40 (m 1H), 3.84 (m 4H), 1.82 (m 8H), 1.65 (m 11H). 13 C NMR ( δ , CDCl 3 ): 156.8 (C), 145.6 (C), 145.4 (C), 144.7 (C), 143.1 (C), 143.0 (C), 142.6 (C), 142.4 (C), 142.3 (C), 142.1 (C), 141.6 (C), 140.1 (C), 120.9 (CH), 66.2 (C), 66.0 (C), 42.2 (CH 2 ), 40.5 (CH 2 ), 40.0 (CH 2 ), 38.2 (CH 2 ), 38.1 (CH 2 ), 37.2 (CH), 36.5 (C), 26.1 (CH). Mass spectrometry: 960 (<1%), 720 (100%), 240 (45%), 202 (100%). High-resolution mass spectrometry: found 961.1632, calculated for C 78 H 24 960.1878. STM experiments Au(111) on mica samples (Agilent) were rinsed with acetone and isopropanol, mounted on a sample holder and transferred to the ultra-high-vacuum preparation chamber. The sample is cleaned by repeated cycles of ion sputtering (2 keV, 15 min) and annealing (540 °C, 45 min). It is then removed to the load-lock chamber under a 5-l min −1 flow of nitrogen gas to minimize backflow of air towards it. A ~100 μl drop of 0.01 mM Dia–C 60 in toluene is deposited on the sample and allowed to spread for 60 s. Before the load-lock chamber is resealed and pumped down, the drop is blown off using nitrogen gas, the sample is rinsed with isopropanol and again blown dry with nitrogen gas. The sample is moved into the STM chamber (pressure below 2 × 10 −11 mbar), and cooled to 4.5 K for observation. STM measurements were typically performed with Pt/Ir (90%/10%) tips. Bias voltage always refers to the sample potential with respect to the tip. I–V spectroscopy is performed by moving the tip to a particular location, turning the feedback loop off and ramping the voltage between the desired values while the current is recorded. dI/dV versus V spectra were collected in a similar fashion and with a lock-in amplifier, with a modulation of few mV added to the bias voltage. Computations DFT computations were performed using the SIESTA code [31] with a double-zeta polarized basis set, GGA (PBEsol) functional and Troullier–Martins pseudopotentials. Atomic structures were allowed to relax until forces were reduced to within 0.05 eV/Å. An energy cutoff of 300 Ry and a uniform 8 × 8 × 1 k -point mesh were used during the computations. STM topographs (at bias voltage V ) were generated by summing the electron density of each eigenstate with energy E between E F and E F +e V . The vibration mode simulations were carried out using a finite difference approach, and an energy cutoff of 1,000 Ry for accurate force constant calculation. How to cite this article: Randel, J. C. et al. Unconventional molecule-resolved current rectification in diamondoid–fullerene hybrids. Nat. Commun. 5:4877 doi: 10.1038/ncomms5877 (2014).